Combinatorial flexibility of cytokine function during human T helper cell differentiation In an inflammatory microenvironment, multiple cytokines may act on the same target cell, creating the possibility for combinatorial interactions. How these may influence the system-level function of a given cytokine is unknown. Here we show that a single cytokine, interferon (IFN)-alpha, can generate multiple transcriptional signatures, including distinct functional modules of variable flexibility, when acting in four cytokine environments driving distinct T helper cell differentiation programs (Th0, Th1, Th2 and Th17). We provide experimental validation of a chemokine, cytokine and antiviral modules differentially induced by IFN-α in Th1, Th2 and Th17 environments. Functional impact is demonstrated for the antiviral response, with a lesser IFN-α-induced protection to HIV-1 and HIV-2 infection in a Th17 context. Our results reveal that a single cytokine can induce multiple transcriptional and functional programs in different microenvironments. This combinatorial flexibility creates a previously unrecognized diversity of responses, with potential impact on disease physiopathology and cytokine therapy. Cytokines are glycoproteins mediating intercellular communication and affecting key cellular functions, such as survival, proliferation and differentiation [1] , [2] . They act through interaction with a cognate receptor expressed on target cells. Because of their pleiotropy, individual cytokines can act on a diversity of cell types, and conversely, one cell type can respond to a diversity of cytokines [1] . This creates the possibility that a cytokine may act on a cell type either alone, or in combination with other cytokines. Complex inflammatory tissue microenvironments are composed of specific sets of cytokines characterizing the inflammatory process. Most studies have focused on the effects of an individual inflammatory cytokine on a given cell type, or have studied combinations of cytokines on a limited number of output responses. When considering the complexity of inflammatory environments, together with the system-level cellular response made of multiple molecular and functional outputs, two important questions arise: (1) could extrinsic factors determine the function of a given cytokine? (2) which part of the large-scale cytokine response would be determined by combinatorial interactions with other cytokines? To address these questions, we used an experimental system combining the following three components: (1) human CD4 T helper (Th) cell differentiation as a system that can be affected by a diversity of cytokines that drive or modulate the differentiation process [3] , [4] , (2) interferon (IFN)-alpha as a cytokine of interest to study its system-level effects using transcriptional profiling and (3) Th cytokine contexts as representative of distinct types of inflammation, that is, Th1, Th2 and Th17, in order to study the effects of IFN in each of these contexts. We selected IFN because it is one of the most pleiotropic cytokines since the IFN receptor is ubiquitously expressed [5] , [6] , [7] , [8] . IFN are widely produced in different types of infection, and also in auto-immunity [9] , [10] , [11] , [12] , [13] , [14] . Hence, IFN act within a diversity of inflammatory contexts characterizing each of these physiopathological conditions. By combining computational and experimental system-level and focused analyses, we demonstrate that a single cytokine can effectively drive a multiplicity of transcriptional signatures in target cells when it functions within specific cytokine environments. IFN-α induces a specific T helper transcriptional signature To address the system-level flexibility of IFN-α function in diverse inflammatory environments, we used CD4 + T helper cell differentiation as a model. Naive CD4 + T cells were cultured for 5 days in the presence of polyclonal stimulation (anti-CD3/CD28) in four distinct polarizing cytokine contexts (Th0, Th1, Th2 and Th17) as previously described [15] , in the presence and absence of IFN-α. Transcriptional profiles were generated using Hugenes ST1.1 Affymetrix chips after 5 days of culture in distinct polarizing conditions, and after 4 h of subsequent restimulation with anti-CD3/CD28 ( Fig. 1a ). These time points mimic two physiological steps in the Th response: (1) the ‘stable’ transcriptional programme occurring during Th differentiation (day 5), (2) the transcriptional programme induced after recognition of the cognate antigen by Th cells (day 5+ 4h restimulation (restim)). First, we focused on the neutral IFN-α signature based on differential gene expression in order to characterize the effects of IFN-α in the unpolarized Th0 condition ( Fig. 1a ). We identified an IFN-α signature comprising 76 and 71 genes, at days 5 and day 5 +4h restim, respectively ( Fig. 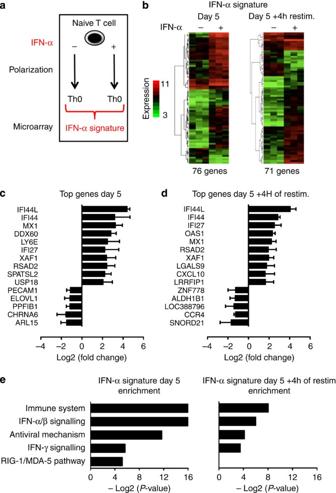Figure 1: IFN-α induces a conserved signature during the differentiation of naive CD4 T cell. (a) Naive CD4 T cells were cultured for 5 days with anti-CD3/CD28 beads in the presence or not of IFN-α. Microarrays chips were hybridized both at day 5 and after 4 h of restimulation with anti-CD3/CD28 beads (day 5 + 4h restim). (b) Hierarchical clustering of the 76 and the 72 genes that represent theIFN-α signatureat both time points.IFN-α signaturewas defined as the IFN-modulated genes in Th0 according to two criteria: fold change (FC)>2 andPvalues<0.05 (pairedT-test). Relative gene expression (log value) of the 15 top induced ofIFN-α signatureat day 5 (c) andIFN-α signatureat day 5 + 4h restim. (d) Data represent the mean (±s.d.) of three independent donors. (e) Enrichment analaysis of theIFN-α signatureat day 5 and day 5 + 4h restim. 1b , Supplementary Table 1 ). Most of the genes were upregulated (55 of 76, and 53 of 71, respectively). Top-induced genes were conserved at both time points, including well-known interferon-stimulated genes (ISGs) such as MX1 , IFI44 , IFI44L , XAF-1 and IFI27 , which mediate the antiviral state in IFN-treated cells ( Fig. 1c,d ). In the IFN-α signature at day 5 +4h restim, we found genes related to chemotactism, such as CXCL-10 (upregulated) and the chemokine receptor CCR4 (downregulated) ( Fig. 1d ). Functional enrichment analysis revealed four modules that were differentially regulated at both time points: immune system, IFN-α/β signalling, antiviral mechanisms mediated by ISGs and IFN-γ signalling ( Fig. 1e ). The RIG-I/MDA-5 induction pathway was statistically significant only at Day 5. These results suggest that IFN confers a specific signature to CD4 + T cells composed of antiviral ISGs that persist even after polyclonal restimulation. Figure 1: IFN-α induces a conserved signature during the differentiation of naive CD4 T cell. ( a ) Naive CD4 T cells were cultured for 5 days with anti-CD3/CD28 beads in the presence or not of IFN-α. Microarrays chips were hybridized both at day 5 and after 4 h of restimulation with anti-CD3/CD28 beads (day 5 + 4h restim). ( b ) Hierarchical clustering of the 76 and the 72 genes that represent the IFN-α signature at both time points. IFN-α signature was defined as the IFN-modulated genes in Th0 according to two criteria: fold change (FC)>2 and P values<0.05 (paired T -test). Relative gene expression (log value) of the 15 top induced of IFN-α signature at day 5 ( c ) and IFN-α signature at day 5 + 4h restim. ( d ) Data represent the mean (±s.d.) of three independent donors. ( e ) Enrichment analaysis of the IFN-α signature at day 5 and day 5 + 4h restim. Full size image IFN-α signature is distinct from Th1, Th2 and Th17 signatures We investigated whether this IFN-α signature was distinct from the Th1, Th2 and Th17 signatures. The Th-specific signatures were defined by differential gene expression between Th0 versus Th1, Th2 and Th17, respectively ( Supplementary Fig. 1a ). We identified 746 differentially expressed genes between the five conditions Th0, Th1, Th2, Th17 and Th0+IFN-α (Methods). We used clustering analysis to evaluate similarities among all the profiles for all donors ( Supplementary Fig. 1b ). Th2 and Th17 profiles were distinct from the Th0, Th1 and IFN-α. Clustering analysis revealed that Th0 and Th1 profiles were more similar to each other than to IFN-α, suggesting that IFN-α induces more variation than IL-12 (used for Th1 differentiation) at the transcriptional level. We compared the IFN-α signature to the specific Th signatures, defined as the differentially expressed genes between the Th0 and each of the specific Th conditions (Th1, Th2 and Th17) ( Supplementary Fig. 1c ). These signatures contained known Th-specific genes, such as IFN-γ in Th1, GATA-3 in Th2, and IL-17F in Th17 ( Supplementary Fig. 2 ), validating the relevance of each signature. We found that the IFN-α signature at day 5 contained a specific set of genes with little overlap with Th1 (12 of 72, 16.7%), Th2 (9 of 133, 6.7%) and Th17 (12 of 236, 5%) signatures, respectively ( Supplementary Fig. 1c ). For example, we found that SPATSL2 and the anti-apoptotic gene CHMP5 were common to the Th2 and Th17 signatures respectively. Only one gene, the integrin PECAM-1 , was decreased by IFN-α as well as in Th1 and Th17 conditions ( Supplementary Fig. 2 ). Our data show that IFN-α induces a unique signature on Th cells distinct from a Th1, Th2 and Th17 signatures, indicating that it does not simply duplicate known effects of standard Th-polarizing cytokines. Flexibility of IFN-α signatures in various Th cytokine contexts Instead of acting alone, as a single agent, IFN is expected to act within diverse cytokine environments, reflecting diverse pathophysiological polarizing contexts. We investigated whether combinatorial stimulation might induce plasticity in the large-scale response to IFN. We compared the neutral IFN-α signature with each of the IFN-α signatures obtained in a Th1, Th2 and Th17 contexts ( Fig. 2a ). Surprisingly, we found that the majority of IFN-modulated genes were dependent on the cytokine context. We identified 65, 67 and 65 genes for the IFN-α signatures in Th1, Th2 and Th17 contexts at day 5, respectively ( Fig. 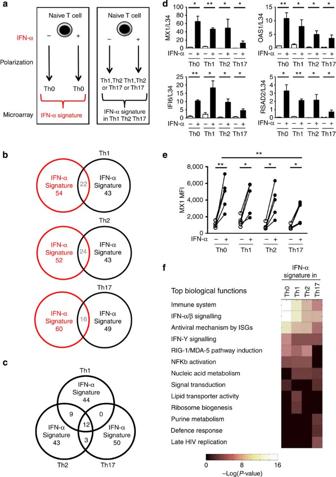Figure 2: T helper inflammatory microenvironments control IFN-α response and generate a diversity of transcriptional and functional programs. (a) Naive CD4 T cells were cultured for 5 days in four different polarizing contexts (Th0, Th1, Th2 and Th17) with anti-CD3/CD28 beads in the presence or not of IFN-α. Microarrays chips were hybridized both at day 5 and day 5 + 4h restim. (b) Venn diagram representing the overlap between theIFN-α signaturein Th0 and the IFN-α signature in the three different polarizing contexts (Th1, Th2 or Th17). For example,IFN-α signaturein Th1 was defined by the genes differentially regulated between Th1+ IFN-α and Th1 according to the following criteria: fold change (FC) >2 andPvalues <0.05 (pairedt-test). (c) Venn diagram representing the overlap between theIFN-αsignaturein the three different polarizing contexts (Th1, Th2 or Th17). (d) Validation of some antiviral genes that belong to the core response of IFN-α (MX1,OAS1,RSAD2andIFI6) by RT-PCR. (e) Mx1 protein was evaluated by intracellular cytokine staining in the eight contexts at day 5. Quantification of Mx1 protein in five donors. (f) Enrichment analysis for theIFN-α signaturein Th0, Th1, Th2 and Th17 at day 5. Data (d,e) represent mean ±s.d. of five independent experiments. *P<0.05; **P<0.01; ns: non-significant (pairedt-test). 2a and listed in Supplementary Table 2 ). The neutral IFN-α signature had less than 30% genes in common with each of the IFN-α signatures in the three Th contexts ( Fig. 2b ). We then quantified the overlap between each of the IFN-α signatures in Th1, Th2 and Th17 ( Fig. 2c ). Only 12 genes were common between the three IFN-α signatures. Most of them (9 out of 12) were known to have an antiviral action. We validated by RT-PCR a stable upregulation induced by IFN-α of four of these genes ( MX1 , OAS1 , IFI6 and RSAD2 ) ( Fig. 2d ). However, the level of induction of these genes was flexible with a lower modulation in Th2 and Th17 environments. We further validated by flow cytometry a similar induction of MX1 by IFN-α at the protein level, in the 4 Th contexts ( Supplementary Fig. 3 and Fig. 2e ). Figure 2: T helper inflammatory microenvironments control IFN-α response and generate a diversity of transcriptional and functional programs. ( a ) Naive CD4 T cells were cultured for 5 days in four different polarizing contexts (Th0, Th1, Th2 and Th17) with anti-CD3/CD28 beads in the presence or not of IFN-α. Microarrays chips were hybridized both at day 5 and day 5 + 4h restim. ( b ) Venn diagram representing the overlap between the IFN-α signature in Th0 and the IFN-α signature in the three different polarizing contexts (Th1, Th2 or Th17). For example, IFN-α signature in Th1 was defined by the genes differentially regulated between Th1+ IFN-α and Th1 according to the following criteria: fold change (FC) >2 and P values <0.05 (paired t -test). ( c ) Venn diagram representing the overlap between the IFN- α signature in the three different polarizing contexts (Th1, Th2 or Th17). ( d ) Validation of some antiviral genes that belong to the core response of IFN-α ( MX1 , OAS1 , RSAD2 and IFI6 ) by RT-PCR. ( e ) Mx1 protein was evaluated by intracellular cytokine staining in the eight contexts at day 5. Quantification of Mx1 protein in five donors. ( f ) Enrichment analysis for the IFN-α signature in Th0, Th1, Th2 and Th17 at day 5. Data ( d , e ) represent mean ±s.d. of five independent experiments. * P <0.05; ** P <0.01; ns: non-significant (paired t -test). Full size image Strikingly, the majority of the IFN-α signature genes were specific to a given Th context, suggesting that ISGs expression that mediates IFN-α function may be driven by diverse cytokine microenvironments. To get a deeper insight into the functions underlying each of the IFN-α signatures in Th0, Th1, Th2 and Th17, enrichment analysis was performed using the Reactome and GO geneset (see Methods). The results confirmed a previously unrecognized flexibility of IFN-α response in a context-dependent manner ( Fig. 2f ). Even if some well-described functions of IFN (for example, antiviral mechanism induced by ISG or RIG-1/MDA5 induction pathway) were conserved across each Th context, their level of induction were dramatically reduced in Th2 and Th17 contexts ( Fig. 2f ). Moreover, the antiviral state induced by IFN was qualitatively and quantitatively reduced in Th17 cells ( Fig. 2c,d ), suggesting that Th subsets may not be equally protected by IFN during viral infection ( Fig. 2d and Supplementary Table 2 ). This flexibility observed in IFN response may be partially explained by differential activation of IFN signalling in Th contexts ( Fig. 2f ). Finally, half of the enriched pathways (6 of 13) were induced by IFN-α only in a single Th context. Among these, IFN-α modulated specifically a biological function related to lipid metabolism only in a Th1 context, and induced pathways related to nucleotide metabolic process and HIV1 transcription process only in a Th17 context, suggesting a different response of IFN-stimulated Th17 cells to HIV-1 infection ( Fig. 2f ). Similar results were obtained with the IFN-α signature at day 5 +4h restimulation ( Supplementary Fig. 4 ). Overall, our analyses at the individual gene and systems levels, revealed an important plasticity of IFN when combined to Th-polarizing cytokines representing diverse inflammatory environments. Context-dependent regulation of the IFN-induced antiviral state Functional analysis of IFN response suggests that the polarizing context influences the antiviral state induced by IFN ( Fig. 2f ). Validation of antiviral ISGs at the RNA level showed quantitative differences among each subset ( Fig. 2d ). Antiviral state was mostly affected in Th2 and Th17 environments. In the latter, we observed a 2–4-fold less induction of RSDA2 and MX1 by IFN-α. This lower Mx1 induction was further confirmed at the protein level ( Fig. 2e and Supplementary Fig. 5a ). To ascertain that the lower induction of MX1 in Th2 and Th17 was not due to an inhibition of Th2 and Th17 cells by IFN-α, we analysed the production of the prototypical Th cytokines IFN-γ, IL-13 and IL-17 in the supernatants in five new independent donors ( Supplementary Fig. 5b ). In our system, IFN-α increased IL-17A in the supernatant of Th17 cells, and inhibited IL-13 in Th2 cells ( Supplementary Fig. 5b ). Thus, the lower Mx1 induction in Th17 cells was not related to an inhibition of Th17 by IFN-α. Finally, the MX1 protein level did not correlate to the level of IFN-γ, IL-13 and IL-17, in Th1, Th2 and Th17 contexts, respectively ( Supplementary Fig. 5c ). We next wondered whether these changes of the antiviral state had a functional impact on Th cells during viral infection. We differentiated distinct Th subsets in the presence and absence of IFN, and infected them with two different GFP-reporter viruses derived from HIV-1 and HIV-2 for 48 h ( Supplementary Fig. 6 ). We observed that Th0, Th1 and Th2 cells differentiated in the presence of IFN were less infected by HIV-2, as compared with an absence of IFN. This IFN-induced protection was dose-dependent (16 versus 32%; 14.8 versus 28.2% and 21.1 versus 37.2% respectively for an MOI of 40) ( Fig. 3a ). However, IFN-α had no significant impact on the protection of Th17 cells ( Fig. 3a ). When Th cells were challenged with our mutant HIV-1, only Th0 and Th1 cells were significantly protected when previously cultured with IFN (17.4 versus 25.6% and 27.2 versus 41.7% respectively) ( Fig. 3b ). 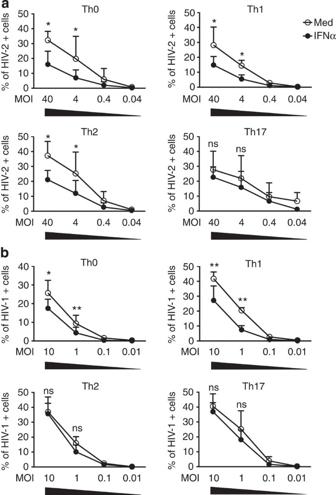Figure 3: Antiviral state induced by IFN-α confers a specific susceptibility to viral infection in a Th subset-dependent manner. Naive T cells were differentiated with anti-CD3 plus anti-CD28 in Th0, Th1, Th2 and Th17 ±IFN-α for 5 days. The same cells were then infected with VSV-G-pseudotyped HIV-1 or HIV-2 viruses expressing GFP (with increasing dose of virus), in the presence of IL-2 for 48H. Infected cells, defined as GFP-positive cells were evaluated by flow cytometry. (a) Infection of Th cells with HIV-2. MOI: multiple of Infection. Data are the mean ±s.d. of five independent experiments. (b) Infection of Th cells with HIV-1. Data are the mean ±s.d. of five independent experiments. NS, non significant, *P<0.05; **P<0.01 (pairedt-test). Figure 3: Antiviral state induced by IFN-α confers a specific susceptibility to viral infection in a Th subset-dependent manner. Naive T cells were differentiated with anti-CD3 plus anti-CD28 in Th0, Th1, Th2 and Th17 ±IFN-α for 5 days. The same cells were then infected with VSV-G-pseudotyped HIV-1 or HIV-2 viruses expressing GFP (with increasing dose of virus), in the presence of IL-2 for 48H. Infected cells, defined as GFP-positive cells were evaluated by flow cytometry. ( a ) Infection of Th cells with HIV-2. MOI: multiple of Infection. Data are the mean ±s.d. of five independent experiments. ( b ) Infection of Th cells with HIV-1. Data are the mean ±s.d. of five independent experiments. NS, non significant, * P <0.05; ** P <0.01 (paired t -test). Full size image Collectively, these data show that the cytokine environment modulated the antiviral response induced by IFN-α in a context-specific manner. This provides a functional level of validation of the combinatorial plasticity of IFN function during Th cell polarization. Environmental control of IFN-induced Th cell polarization Most of the context-dependent functions of IFN-α were related to RNA and DNA metabolism, which controls transcription and replication. However, we also found genes related to immune functions that characterize Th cells. In order to get a deeper insight, we defined four main « modules » related to the top biological functions that characterize Th cells: cytokine, transcription factor, chemokine and receptor. We identified within all four IFN signatures (Th0, Th1, Th2 and Th17), the ISGs that were involved in these four modules in view of further functional validation ( Supplementary Table 3 ). Analysis of the IFN-α signature in Th1, Th2 and Th17 revealed that IFN regulated specific components of the chemokine and receptor module in a context-dependent manner (CXCL10 in Th1, CCL20 in Th17, CCR4 in Th0). Microarray data were validated at the protein level for chemokine ligand/receptor pairs including, CXCL10 in Th0 and Th1, as well as CCR4 in Th0 and Th1 and finally CCL20 in Th17 ( Fig. 4a,b ). The results obtained here confirm that IFN induced a specific chemokine secretion pattern dictated by the Th cytokine environment. 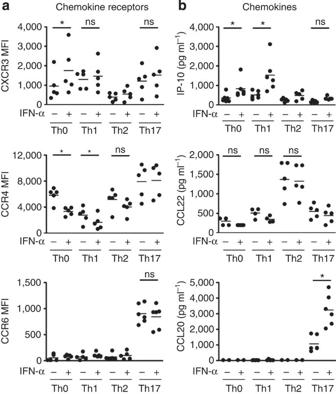Figure 4: IFN-α modulates specifically the chemokine/chemokine receptor of each Th subset. ELISA, cytometric bead assay and flow cytometry analysis of (a) CXCR3, CCR4 and CCR6 (b) IP-10, CCL22 and CCL20. CD4 T cells were polarized in Th0, Th1, Th2 and Th17 cells with anti-CD3/CD28 beads in the presence or absence of IFN-α for five days. Cells were re-stimulated with anti-CD3/CD28 beads. Flow cytometry was performed after 12 h. Supernatants were collected after 24 h for chemokine analysis. ND, non-detectable; *P<0.05; **P<0.01 (Wilcoxon test (N>6) or Student’st-test (N<6)). Data represent five to six independent experiments. Figure 4: IFN-α modulates specifically the chemokine/chemokine receptor of each Th subset. ELISA, cytometric bead assay and flow cytometry analysis of ( a ) CXCR3, CCR4 and CCR6 ( b ) IP-10, CCL22 and CCL20. CD4 T cells were polarized in Th0, Th1, Th2 and Th17 cells with anti-CD3/CD28 beads in the presence or absence of IFN-α for five days. Cells were re-stimulated with anti-CD3/CD28 beads. Flow cytometry was performed after 12 h. Supernatants were collected after 24 h for chemokine analysis. ND, non-detectable; * P <0.05; ** P <0.01 (Wilcoxon test ( N >6) or Student’s t -test ( N <6)). Data represent five to six independent experiments. Full size image We next focused on the cytokine module, which represents the most characterized function of Th cells. Among Th-derived cytokines, only IFN-γ was upregulated in the IFN-α signature at the mRNA level in a Th1 and Th17 environment ( Supplementary Table 3 ). However, considering the difference in kinetics of transcription, post-transcriptional modifications and/or secretion of different Th cytokines, we anticipated that other Th cytokines might be modulated by IFN-α at the protein level. To better clarify the role of IFN-α on Th cytokine secretion, we measured the protein levels of 14 different Th-derived cytokines in the supernatant 24 h after restimulation by ELISA and CBA, in the same priming conditions as were used for the transcriptional studies. The prototypical Th cytokines IFN-γ, IL-4, IL-17 and IL-10 were modulated by IFN-α in a context-dependent manner ( Fig. 5a ). IFN-γ was significantly and specifically increased in Th1 and Th17 conditions. IL-4 secretion was inhibited by IFN-α only in Th0 and Th2 environments, without concomitant inhibition of GATA-3 ( Supplementary Fig. 7 ). Moreover, Th2 cells increased specifically IL-10 secretion, without modification in FoxP3 nor c-MAF mRNA. Surprisingly, we found that IFN-α also increased RORc expression and IL-17 production but only in a Th17 context ( Fig. 5a and Supplementary Fig. 7 ). 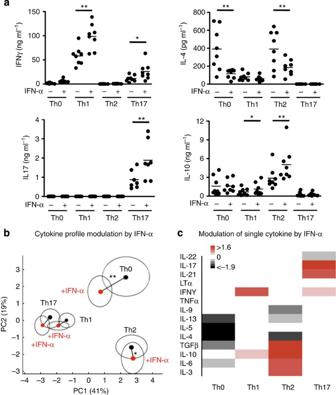Figure 5: IFN-α has a context-dependent effect on the cytokine profile of each Th subset by modulating set of cytokines. Naïve T cells were differentiated with anti-CD3/CD28 in Th0, Th1, Th2 and Th17 ±IFN-α for 5 days and re-stimulated for 24 h with anti-CD3/CD28 to collect supernatant. (a) ELISA and/or cytometric bead assay of IL-4, IL-17, IL-10 and IFN-γ in supernatants. *P<0.05; **P<0.01 (Wilcoxon test). Data are the mean of eight independent experiments. (b) PCA of the 14 Th-related cytokines (IL-3, IL-4, IL-5, IL-6, IL-9, IL-10, IL-13, IL-17, IL-21, IL-22, IFN-γ, TNF-α, LT-α and TFG-β) in eight experimental conditions: Th0, Th1, Th2, Th17 ±IFN-α. Points represent the mean of all values for six donors. Ellipses represent the s.d. for each condition along the principal components analysis. The red line represents the ‘shift’ of the Th profile. A MANOVA test was applied to discriminate statistical difference between the global cytokine profiles *P<0.05; **P<0.01 (MANOVA test). (c) Heatmap represents the modulation of individual cytokine secretion by IFN-α in the 4 Th contexts. Red represents increased and black decreased values. Fourteen cytokines were measured by ELISA and/or CBA. For each cytokine, the mean value obtained from six individuals donors was normalized (centre and reduced) in all eight conditions. Modulation was then defined by difference (Δ) of the normalized data according to the presence or absence of IFN-α. Figure 5: IFN-α has a context-dependent effect on the cytokine profile of each Th subset by modulating set of cytokines. Naïve T cells were differentiated with anti-CD3/CD28 in Th0, Th1, Th2 and Th17 ±IFN-α for 5 days and re-stimulated for 24 h with anti-CD3/CD28 to collect supernatant. ( a ) ELISA and/or cytometric bead assay of IL-4, IL-17, IL-10 and IFN-γ in supernatants. * P <0.05; ** P <0.01 (Wilcoxon test). Data are the mean of eight independent experiments. ( b ) PCA of the 14 Th-related cytokines (IL-3, IL-4, IL-5, IL-6, IL-9, IL-10, IL-13, IL-17, IL-21, IL-22, IFN-γ, TNF-α, LT-α and TFG-β) in eight experimental conditions: Th0, Th1, Th2, Th17 ±IFN-α. Points represent the mean of all values for six donors. Ellipses represent the s.d. for each condition along the principal components analysis. The red line represents the ‘shift’ of the Th profile. A MANOVA test was applied to discriminate statistical difference between the global cytokine profiles * P <0.05; ** P <0.01 (MANOVA test). ( c ) Heatmap represents the modulation of individual cytokine secretion by IFN-α in the 4 Th contexts. Red represents increased and black decreased values. Fourteen cytokines were measured by ELISA and/or CBA. For each cytokine, the mean value obtained from six individuals donors was normalized (centre and reduced) in all eight conditions. Modulation was then defined by difference (Δ) of the normalized data according to the presence or absence of IFN-α. Full size image It is known that Th cells produce a broad array of cytokines, which contribute to the global Th responses [15] . Whether IFN-α is able to modulate the global cytokine profile of each Th cells, and to what extent such a function may be affected by combinatorial plasticity is not known. To address this issue, we used principal component analysis (PCA) as a dimensionality reduction method to analyse the full data set of fourteen cytokines in eight culture conditions addressing the effects of IFN in Th0, Th1, Th2 and Th17 contexts ( Fig. 5b ). Each point of the PCA plane represents the reduction in two dimensions of the 14-dimensional cytokine profiles. IFN-α determined a shift of the cytokine profiles (as defined by the direction and the length of the vectors) that differed in Th0, Th1, Th2 or Th17 environments ( Fig. 5b ). PCA confirmed the context-dependent effect of IFN-α on the cytokine profile in each Th environment. Only the modulation of the Th0 and Th2 global profiles by IFN-α was statistically significant according to a multivariate ANOVA (MANOVA) test ( Supplementary Fig. 8 ). However, this did not exclude significant changes at the individual cytokine level. Next, we investigated whether the change in the global cytokine profile was due to modulation of a single or multiple cytokines. We found that IFN-α modulated a specific set of cytokines in each polarizing context ( Fig. 5c ). In a Th1 environment, IFN increased IFN-γ and to a lesser extent IL-10. In a Th2 environment, IFN inhibited IL-4, IL-9 and IL-13, while increasing IL-10, IL-6, IL-3 and TGF-β. Finally, Th17 modulation was explained by an increase in IL-17, IL-21 and IFN-γ, and an inhibition of IL-22 ( Fig. 5c ). Overall, the system-level context-dependent effects of IFN-α were confirmed at the protein level within the chemokine and cytokine modules. These results also validated the concept that the immune-modulating functions of IFN are highly flexible, including the most conserved antiviral functions, as evidenced by the analysis of multiple IFN signatures. Our study reveals a previously unsuspected system-level flexibility in IFN-induced transcriptional programs depending on the Th-polarizing cytokine context, with a validated functional impact. We propose the concept of combinatorial flexibility as the ability of a given cytokine to induce a diversity of large-scale responses, and associated functional states, when acting in combination with other cytokines. By using a system-level approach, we found that combinatorial flexibility leads to distinct qualitative and quantitative IFN signatures, with the majority of the gene sets being specific to a given Th context. An important question was the functional consequences of the combinatorial flexibility. Type I IFN are pleiotropic cytokines, with highly conserved antiviral functions across evolution [16] , [17] . Our study revealed a previously unrecognized flexibility of the IFN-induced antiviral response. The antiviral ISGs expression was similar in Th0 and Th1, but decreased in Th2 and mainly Th17 contexts. This led to reduced protection of Th cells during HIV infection in a Th17, as compared with Th0 or Th1 contexts. Previous reports have shown that Th17 cells were reduced either in blood or in the lamina propria of HIV-1-infected patients [18] , [19] . Thus, the ‘lower’ antiviral state induced by IFN during HIV infection may contribute to this phenomenon. A combination of ISGs is required to obtain a strong and complete control of virus replication [20] . In our system, the quantitative difference of expression in many ISGs may explain the flexibility of the antiviral response in different Th contexts. Besides cell-intrinsic antiviral functions, IFNs have adjuvant effects on immune cells [5] , [7] , [8] . We showed that functional flexibility was also observed among Th-specific functions, such as cytokine or chemokine module, which was validated at the protein level ( Fig. 4 ). In the latter, the most striking result was observed for CCL20, which was greatly and only enhanced by IFN in a Th17 context. To our knowledge, this is the first report of secretion of CCL20 in human Th17 cells, indicating that combinatorial plasticity may lead to emerging functions. CCL20 is known to attract CCR6+ cells, including Th17 cells and have a critical role in Th17 cells homeostasis [21] . Thus, CCL20 and IL-17 upregulation by IFN in a Th17 context may serve as a mechanism to amplify pre-existing Th17 responses. Large-scale combinatorial flexibility may also reconcile some paradoxical or controversial results on a given cytokine. Context-dependent effects may be overlooked when comparing results from different studies. For example, IFN is often described as a ‘Th1 dominant’ cytokine even if not sufficient to induce a stable Th1 phenotype [22] . Further studies emphasized this property as IFN inhibited both human and mice Th2-driven polarization [23] or Th17-driven polarizaton [24] , [25] . However, recent studies raised the question of a ‘unique’ effect of IFN on Th cells. IFN was able to maintain human Th17 phenotype [26] , increase human Th9 differentiation [27] and induced in the presence of IL-10 a regulatory phenotype in mice [28] . Part of the ongoing controversy may be due to the comparison of Type I IFN effects in different contexts. In our study, we performed a systematic analysis in all major Th cytokine differentiation conditions (Th1, Th2 and Th17), and analysed a diversity of effector Th output cytokines, instead of restricting our study to a given Th subset. In this manner, we could dissect the variability in IFN responses, and associate it to specific sets of input and output Th cytokines. Our findings are also consistent with recent data emphasizing the critical role of commensal bacteria in controlling systemic antiviral immunity [29] , [30] , [31] , [32] . It has been shown that commensal-derived signals are capable of limiting or exacerbating infection in the intestinal microenvironment. The mechanisms involved are diverse, either by contributing to DC maturation and subsequent T-cell priming in the lung [29] , or increasing responsiveness to virus by modulating their threshold of activation, as described with macrophages [32] . Moreover, a tonic microbiota is mandatory for optimal lymphotoxic function of CD8+ T cells and natural killer cells during viral infection. Conversely, commensal infection can increase chronic viral infectivity in the gastrointestinal microenvironment through cytokine modulation [30] , [31] . Finally, certain gut bacteria affect differentially Th cell polarization: Segmented filamentous bacteria induce Th17 cells, whereas Clostridium species induce regulatory T cells in the colon [33] , [34] , [35] . Taken together, our results suggest an additional mechanism that may contribute to the microbiota-regulated type I IFN response in priming for different types of inflammatory and immune responses. A detailed understanding of the effects of a cytokine is particularly important in cytokine therapy. Our results revealed a new level of complexity in IFN responses, which may also explain the diversity of IFN responses in therapeutics [5] . IFN are used to treat a variety of auto-immune, infectious and neoplastic diseases, most important of which are hepatitis C, multiple sclerosis and malignant melanoma [5] , [36] , [37] , [38] . Our results suggest that each disease-specific inflammatory environment (extrinsic factors) may drive a specific IFN response, which may underlie the diversity of effects observed with therapeutic IFN. Although established in human Th cells, the same conceptual and methodological framework may be applied to dissect the function of other cytokines and soluble factors in contexts associated with a given physiopathological situation. We can anticipate that a diversity of functional outputs may be observed, which would change our interpretation of cytokine function by attributing a large part to the context rather than to the nature of the cytokine itself. Given the number of possible combinations within an inflammatory microenvironment, and their expected impact on cytokine function, our findings may have a broad impact through the precise characterization of their large-scale combinatorial flexibility. Purification of naive CD4+ T lymphocytes from adult blood Peripheral blood mononuclear cells were separated by Ficoll–Hypaque centrifugation (Amersham Biosciences) from buffy coats obtained from healthy donors (Saint Antoine-Crozatier Blood bank, Paris). All cells were used with the approval of the Institutional Review Board of Institut Curie, and blood donors gave their informed consent for research use of buffy coats in accordance with the Declaration of Helsinki. CD4 + T lymphocytes were then purified by immunomagnetic depletion with the human CD4 + T cell Isolation Kit II (Miltenyi Biotec), followed by staining with allophyco-cyanin-anti CD4 (clone VIT4 (1/80); Miltenyi Biotec), phycoerythrin-anti-CD45RA (clone HI100 (1/20); BD Bioscience), fluorescein-isothiocyanate-anti-CD45RO (clone UCHL1 (1/20); BD Bioscience) and phycoerythrin-7-anti-CD25 (clone MA-251 (1/20); BD Bioscience). Naive CD4 + T cell sorting of CD4 + CD45RA + CD45RO − CD25 − had a purity of over 99% with a FACSAria (BD Bioscience). T helper cell differentiation assay Naive CD4 + T cells were cultured in 48-well plates (Falcon) at a density of 8 × 10 4 cells per well in X-VIVO 15 serum-free medium (Lonza) in the presence of Dynabeads CD3/CD28 T cell expander (Invitrogen) and polarized into Th0, Th1, Th2 and Th17 with the following cytokines: none for Th0; IL-12 (10 ng ml −1 ; R&D Systems) for Th1; IL-4 (25 ng ml −1 ; R&D Systems) for Th2; IL-1β (10 ng ml −1 ; Peprotech), IL-6 (20 ng ml −1 ; Peprotech), IL-23 (100 ng ml −1 ; R&D Systems) and TGF-β (1 ng ml −1 ; Peprotech) for Th17. IFN-α (Miltenyi) was added at 10 ng ml −1 . After 5–6 days, cells were collected and washed extensively. Cells were re-stimulated at a density of 1 × 10 6 cells per ml for 24 h (for ELISA, Cytometry Beads Array CBA and RT-PCR). Analysis of cytokine and chemokine production The following cytokines and chemokines were measured in culture supernatants by ELISA: IL-17 and IL-22 (R&D System), IL-21 (eBioscience), CCL20 (R&D System). IL-3, IL-4, IL-5, IL-6, IL-9, IL-10, IL-13, IFN-γ, TNF-α, LT-α, TFG-β and CXCL10 were measured by CBA (BD Bioscience) according to the manufacturer’s instructions. Intracellular and surface staining For surface markers cells were stained by incubation for 15 min on ice with the corresponding fluorescence-labelled antibodies: phycoerythrin anti-CCR6 (clone 11A9 (1/40); BD Bioscience), AlexaFluor647 anti-CCR4 (clone TG6/CCR4 (1/80); Biolegend) and AlexaFluor647 anti-CXCR3 (clone G025H7 (1/40); Biolegend). For the detection of Mx1 protein, cells were stained with the live/dead kit (Invitrogen) for 30 min at 4 °C, then fixed with the IC fixation buffer (eBioscience), permeabilized for 45 min at 21 °C with the permeabilization buffer (eBioscience). Cells were stained for 30′ at 21 °C with a primary Rabbit antibody against Mx1 (Clone ab95926, (1/250); Abcam), washed and stained with a secondary antibody (donkey anti rabbit cy5, (1/100); Jackson Immunoresearch). Virus production and infection of CD4+T cells Three different plasmids were used: HIV-GFP (NL4-3 Δ vif Δ vpr Δ vpu Δ env Δ nef with the GFP open reading frame in place of nef ), HIV-2 ROD9 Δenv GFP (ROD9 Δ env Δ nef with the GFP open reading frame in place of nef ), and CMV-VSVG have been described previously [39] . Viral particles were produced by transfection of 293FT cells with 3 μg DNA and 8 μl TransIT-293 (Mirus Bio); for HIV1-GFP, 0.4 μg CMV-VSVG and 2.6 μg HIV-GFP; for HIV2-GFP, 0.4 μg CMV-VSVG and 2.6 μg HIV-2 ROD9 Δenv GFP. One day after transfection, media was removed, cells were washed out once and fresh media was added. Viral supernatants were harvested 1 day later and debris were removed by using a 0.45-μm syringe filter. Virus titres were measured on GHOST X4R5 cells titration as previously described [39] ; briefly, 5 × 10 3 GHOST cells were infected with serial dilutions of HIV-GFP(G) in 200 μl. At 48 h after infection, the proportion of infected GHOST cells was measured by flow cytometry. The viral titration curve was determined on GHOST cells and used to calculate MOI for infection of T cells. At day 5 of naive T cell differentiation, cells were harvested, counted and resuspended in fresh media at the concentration of 1 million per ml with 8 μg ml −1 protamine and 100 μl was aliquoted in round-bottomed 96-well plates. For infection, 100 μl of media or dilution of virus supernatants were added. Forty-eight hours after infection, cells were fixed using 1% paraformaldehyde and GFP-positive cells were evaluated by FACSVerse (BD). Real-time quantitative RT-PCR Total RNA was extracted by RNeasy Micro kit (Qiagen) and processed as previously described [15] . The following probes (Applied Biosystems) were used: FoxP3 (Hs00203958_m1), GATA-3 (Hs00231122_m1), T-bet (Hs00203436_m1), RORc (Hs01076112_m1), AHR (Hs00169233_m1) and c-Maf (Hs00193519_m1). For each sample, mRNA abundance was normalized to the amounts of ribosomal protein L34 (Hs00241560_m1). Affymetrix microarray hybridization Microarray analyses were performed at two time points: either before restimulation (day 5) or four hours after restimulation (day 5 + 4H restim). For each condition, 500 pg of RNA were used to synthesize targets using the WT-Ovation Pico RNA amplification system (Nugen, Bemmel, the Netherlands). Labelled DNA was hybridized on the Affymetrix human Gene ST1.1, processed on an Affymetrix GeneTitan device. The data are derived from three independent donors. Statistical analysis and data mining A nonparametric two-tailed Wilcoxon test or a Student’s t -test was used for pair-wise comparisons of cytokines. MANOVA test was used for comparison of the Th cytokine profile. P values of ≤0.05 were considered statistically significant. We used the Pearson correlation coefficient to assess the significance of correlation between MX1 and IFN-γ, IL-13 and IL-17 The microarray data derived from three independent experiments were normalized using the RMA algorithm and bioinformatics analysis was performed using GeneSpring GX 7.3 (Agilent, Palo Alto, CA, USA) or EMA (Bioinformatique, Institut Curie) on R software [40] . Probes with a signal <20 were excluded. For IFN-α signature, differential gene expression was defined according to the two following criteria: fold change >2; P value <0.05 (paired t -test). Data for the clustering and PCA were processed and analysed as previously described [15] . The Euclidean correlation distance and the Ward’s criteria as an agglomerative method were used for hierarchical clustering analysis. To analyse the genes differentially expressed among Th0, Th0+IFN-α, Th1, Th2 and Th17, we selected the genes according to the following criteria: ANOVA Test with a Tukey HSD test P <0.05 and a false discovery rate (Benjamini–Hochberg) P <0.05. Functionnal analysis were performed using the Molecular Signatures Database (MSigDB). Reactome and GO genes set were used to compute overlap with each IFN signature with a FDR q value below 0.3. Accession codes : The microarray data have been deposited in Gene Expression Omnibus database under accession code GSE 54627 . How to cite this article: Touzot, M. et al. Combinatorial flexibility of cytokine function during human T helper cell differentiation. Nat. Commun. 5:3987 doi: 10.1038/ncomms4987 (2014).